Geometrically protected reversibility in hydrodynamic Loschmidt-echo experiments When periodically driven, a number of markedly different systems (colloids, droplets, grains, flux lines) have revealed a transition from a reversible to an irreversible dynamics that hardly depends on the very nature of the interacting objects. Yet, no clear structural signature has been found for this collective self-organization. Here, we demonstrate an archetypal Loschmidt-echo experiment involving thousands of droplets that interact in a reversible fashion via a viscous fluid. First, we show that periodically driven microfluidic emulsions self-organize and geometrically protect their macroscopic reversibility. Self-organization is not merely dynamical: it has a clear structural signature. Second, we show that, above a maximal shaking amplitude, structural order and reversibility are lost simultaneously through a first-order non-equilibrium phase transition. We account for this discontinuous transition in terms of a memory-loss process. Finally, we suggest potential applications of microfluidic echo as a robust tool to tailor colloidal self-assembly at large scales. The echo protocol consists in studying the evolution of a system after a reversal in its dynamics. Both from a theoretical and an applied perspective, echo protocols have attracted much interest in fields as diverse as quantum information [1] , medical imaging, high T c superconductors [2] , fluid mechanics [3] , granular [4] and soft matter [5] , [6] , [7] , [8] . For instance, in statistical and nonlinear physics, the echo dynamics of chaotic systems has been an area of intense fundamental research since the original debate between Loschmidt and Boltzmann about the emergence of macroscopic irreversibility in systems governed by time-reversible laws at the microscopic level [9] . Conversely, in the condensed matter and mechanics communities, the echo protocols had been predominantly used as effective characterization methods (for example, neutron and NMR spin echo) until publication of a seminal set of experiments by Pine et al. [6] , [10] These experiments consist in shearing periodically a concentrated suspension, in which actual irreversible collisions overcome the reversible hydrodynamic interactions between the particles [10] , [11] . Unexpectedly, it was found that when decreasing the driving amplitude the system self-organizes and displays a bona fide non-equilibrium second-order transition, yielding a macroscopically reversible state. The authors hence revealed a behaviour somehow opposite to Loschmidt’s gedanken experiment, suggested 137 years ago [1] , [9] : macroscopic reversibility emerges from an underlying time-irreversible dynamics. A surge of theoretical studies then showed that the irreversible-to-reversible transition belongs to the universality class of directed percolation [10] , [12] , [13] , thereby identifying reversibility as the trapping in an absorbing state. In addition, subsequent experiments showed that this scenario is relevant to a broader class of classical many-body systems including driven vortices in type-II superconductors [2] and dense granular media [4] . Notably, until now, no structural change has been observed at the irreversible-to-reversible transition, and this phenomenon has been referred to as a ‘random self-organization’. Here we introduce an archetypal Loschmidt-echo experiment. We take advantage of a microfluidic setup in which more than N ~2 × 10 5 interacting droplets evolve according to a time-reversible dynamics at the microscopic level. This setup makes it possible to probe the emergence of macroscopic irreversibility from the single particle to the entire system level, as the droplets are driven in a periodic fashion. We first provide a quantitative definition of the system reversibility, which does not depend on the resolution of the measurement apparatus. We then demonstrate that macroscopic irreversibility arises only above a minimal driving amplitude, in the form of a first-order non-equilibrium phase transition. Conversely, in the small driving regime we demonstrate that structural order emerges in the emulsion and geometrically protects reversible macrostates. This spatial ordering corresponds to the formation of two coexisting liquid-like phases. The simultaneous loss of reversibility and translational order at higher drivings is then explained by investigating how this many-body system forgets about its trajectory on periodic driving. We conclude our article by discussing practical applications of these fundamental results, with a special emphasis on large-scale colloidal self-assembly. A microfluidic echo experiment The experimental setup is thoroughly described in the Methods section. The system is composed of spherical oil droplets dispersed in an aqueous solution ( Fig. 1a ). This emulsion is confined in a 5-cm-long and 5-mm-wide microchannel shown in Supplementary Fig. 1 . The droplets are highly monodisperse, their diameter a =25.5±0.5 μm is comparable to the channel height h =27±0.1 μm. In all that follows the area fraction is set to φ =0.36±0.02. We use a high-precision syringe pump to drive the oil droplets in a periodic fashion, see Fig. 1a and Supplementary Movie 1 . The instantaneous water flow rate is sinusoidal: Q ( t )= Q sin(2 πt / T ), where T is the actuation period. The experiment consists in tracking the instantaneous position ( x i ( t ), y i ( t )) of ~3,000 droplets at the centre of the channel over hundreds of oscillation periods. Already over a single period, the long-range hydrodynamic interactions between the droplets alter their motion [14] . The trajectories fluctuate around the straight lines parallel to the x axis that passive tracers would follow ( Fig. 1a ). However, the centre of mass of the particles displays a well-defined periodic motion along the x direction, with a residual drift one order of magnitude smaller than the smallest driving amplitude. Defining the instantaneous mean particle displacement δ ( t )≡‹ x i ( t )− x i ( t =0)› i , we find that δ ( t ) oscillates in a sinusoidal manner at a period T with an amplitude Δ that scales as QT , see Fig. 1b . Within our experimental conditions, δ ( t ) deviates by less than 5% from an ideal sinusoidal trajectory. We shall also note that the droplets might undergo minute displacements in the z direction (at most 1.5 μm). The resulting relative change in their longitudinal velocity would be as small as 10 −3 . In addition, a sole two-dimensional (2D) description of the droplet motion has proven to yield excellent agreement with experiments in DC flows [14] . Therefore, we disregard potential droplet flutuations in the z direction. 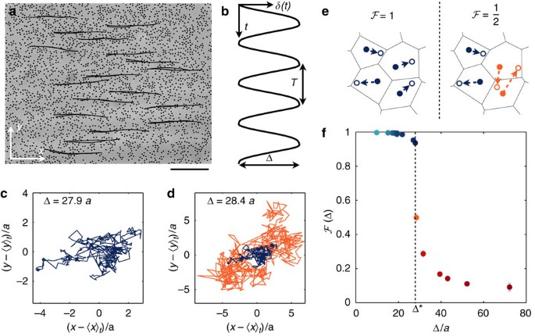Figure 1: Particle trajectories and fidelity loss. (a) Typical snapshot of an experiment. Eighteen single-cycle trajectories are superimposed (black lines). Scale bar: 500 μm. (b) Variations of the instantaneous mean displacementδ(t)≡‹xi(t)−xi(t=0)›iplotted versus time over four cycles.δ(t) oscillates at a periodTwith an amplitude Δ. Here, Δ=27.9aandT=10 s. Average performed over ~3,000 trajectories. (c) Strobed trajectory followed by a single particle over 500 cycles (driving amplitude, Δ1=27.9a). (d) Orange curve: Strobed trajectory followed by a single particle over 500 cycles (driving amplitude, Δ2=28.4a). Blue curve: same trajectory as in (c). (e) Schematic picture to guide the definition of the fidelity function . The positions of four droplets at the beginning of the cycle (filled circles) define the Voronoï cells. In the left panel, all four droplets return to their initial Voronoï cells at the end of the cycle (empty circles), which corresponds to =1. In the right panel, only two droplets return to their initial cells (blue circles). The two others escape after a cycle (red circles). This case corresponds to =0.5. (f) Evolution of the fidelity with the driving amplitude Δ. The colour of the markers codes for Δ, same colour code throughout the entire document. The error bars corresponding to the standard deviation are smaller than the marker size. A threshold amplitude Δ* is clearly defined: below Δ*, remains close to 1, while above the fidelity decays sharply. Figure 1: Particle trajectories and fidelity loss. ( a ) Typical snapshot of an experiment. Eighteen single-cycle trajectories are superimposed (black lines). Scale bar: 500 μm. ( b ) Variations of the instantaneous mean displacement δ ( t )≡‹ x i ( t )− x i ( t =0)› i plotted versus time over four cycles. δ ( t ) oscillates at a period T with an amplitude Δ. Here, Δ=27.9 a and T =10 s. Average performed over ~3,000 trajectories. ( c ) Strobed trajectory followed by a single particle over 500 cycles (driving amplitude, Δ 1 =27.9 a ). ( d ) Orange curve: Strobed trajectory followed by a single particle over 500 cycles (driving amplitude, Δ 2 =28.4 a ). Blue curve: same trajectory as in ( c ). ( e ) Schematic picture to guide the definition of the fidelity function . The positions of four droplets at the beginning of the cycle (filled circles) define the Voronoï cells. In the left panel, all four droplets return to their initial Voronoï cells at the end of the cycle (empty circles), which corresponds to =1. In the right panel, only two droplets return to their initial cells (blue circles). The two others escape after a cycle (red circles). This case corresponds to =0.5. ( f ) Evolution of the fidelity with the driving amplitude Δ. The colour of the markers codes for Δ, same colour code throughout the entire document. The error bars corresponding to the standard deviation are smaller than the marker size. A threshold amplitude Δ* is clearly defined: below Δ*, remains close to 1, while above the fidelity decays sharply. Full size image Δ is the sole control parameter of our echo experiments: starting from the same initial conditions, we investigate the global reversibility of the droplet trajectories as Δ is increased. We stress that we henceforth focus on the long-time dynamics of the periodically driven emulsions, where all the measured quantities have reached their stationary value. Fidelity decay in shaken emulsions Supplementary Movies 2,3 show the dynamics of the droplets for two different, but very close, driving amplitudes Δ 1 =27.9 a and Δ 2 =28.4 a , respectively. These two movies are strobed at a period T . In Supplementary Movie 2 , the particles merely fluctuate around their initial position. It is therefore possible to keep track of each particle by inspecting their strobed pictures only. Increasing Δ by 2% only yields a markedly different dynamics. In Supplementary Movie 3 , the strobed trajectories are composed of apparently uncorrelated large amplitude jumps, which prohibit tracking the individual droplet positions. This significant qualitative change in the strobed trajectories suggests that the system undergoes a sharp transition from a reversible to an irreversible state. Let us now provide a quantitative description for this intuitive picture. The strobed trajectory of a single droplet is shown in Fig. 1c (resp. d) for Δ 1 (resp. Δ 2 ). Irrespective of the driving amplitude, they look like random walks. Strictly speaking none of the two dynamics is reversible, as even for the smaller amplitude the strobed trajectory does not amount to a single point. Therefore, the distinction between the two dynamics is intrinsically related to the spatial resolution at which we observe them, see Fig. 1c,d . To minimize the impact of spatial resolution, we quantify the amount of reversibility without referring explicitly to the magnitude of the particle displacements. Here a system is defined to be reversible if the particle positions can be inferred solely from the inspection of two subsequent strobed pictures. The weakest constraint on the trajectories to solve this inference problem in a unambiguous fashion is that the particles at t + T do not escape the Voronoï cell they occupied at t . Any algorithm based on distance minimization would indeed fail in reconstructing deterministically the droplets’ trajectory if this topological condition was not met. As exemplified in Fig. 1e , we introduce the fidelity function (Δ), which is the time-averaged fraction of droplets that occupy the same Voronoï cell at the beginning and at the end of a period. A perfectly reversible dynamics corresponds to =1, whereas a fully irreversible system is characterized by =0. This definition reflects our initial intuitive criteria. We recall here that is a stationary quantity reached after a number of oscillations. We may note that, not surprisingly, is an overlap function between two conformations of the system akin to that defined in [15] , [16] to quantify dynamical heterogeneities in amorphous granular ensembles. Irreversibility as a breakdown of self-organization The variations of (Δ) are plotted in Fig. 1f . remains close to at small amplitudes. Above a well-identified threshold: Δ*/ a =28.1±0.3, the fidelity decays sharply towards very small values and plateaus as Δ is further increased. Increasing Δ by 2% around Δ*, the number of droplets remaining in their Voronoï cell drops from 94 to 50%. The extreme sharpness of the fidelity loss is a strong hint of a genuine non-equilibrium phase transition. Two comments are in order. First, the strong fidelity decay is all the more surprising insofar, as the droplets interact almost exclusively via reciprocal flows. The capillary number, Ca, that quantifies how much the droplets are deformed by the flow gradients is indeed kept below Ca=10 −4 in all our experiments. Accordingly, we observe no change in the drop shape in the course of a cycle. The Reynolds number, Re, is also much smaller than 1 both in the oil and in the water phases: Re<10 −2 . In addition, during half a cycle, the fluid momentum diffuses over a distance that scales as , where η is the water viscosity and ρ its density, within our experimental conditions ℓ ~3 mm, which is comparable to the channel width. Consequently, the fluid flows in the two phases are very well accounted for by the Stokes equation, which is invariant under time reparametrization [17] . In addition, we stress that the droplets only experience lubricated contacts with the other droplets and the walls. Actual contacts would result in coalescence or wall-wetting events. None of these events were observed in the entire ensembles of ~2 × 10 5 droplets. Altogether, these four observations imply that the droplets are chiefly coupled by time-reversible hydrodynamic interactions at all inter-particle distances. We can thus already conclude that any macroscopic fidelity loss must arise from the collective amplification of minute irreversible processes that cannot be probed at the single/two particle levels. A second important comment is that the uniform flow field in the aqueous phase does not provide any intrinsic length scale to set the value of Δ*. This situation contrasts with the previous mechanical echo experiments, which are all based on a macroscopic shear deformation [4] , [6] , [8] . The non-uniformity of shear flows yields a natural criterion for the ‘critical’ strain amplitude, γ , at which particle collisions occur. The fidelity decay is then expected to occur when the relative displacement γa between two particles moving along two parallel flow lines separated by a equals the typical inter-particle distance (in ). In our Hele–Shaw geometry, the mean flow is a plug flow that can merely advect the droplet ensemble in a uniform fashion. This observation further supports the hypothesis that the hydrodynamic interactions are responsible for the transition towards a macroscopically (ir)reversible state in our experiments. To gain a deeper physical insight in the collective nature of this discontinuous phase transition, we quantify how much the system differs from its initial conformation in the course of a cycle. We introduce an ‘instantaneous’ fidelity function F Δ ( T , T + t ) where t ε[0, T ], which is defined as the fraction of droplets that occupy the same Voronoï cell at time t as at the beginning of a cycle. (The positions of the droplets are measured in the frame of the centre of mass of the N droplets to discard trivial advection.) We show the variations of F Δ ( T , T + t ) averaged over 15 cycles as a function of the instantaneous mean displacement δ ( t ) in Fig. 2a where the colour codes for the driving amplitude. 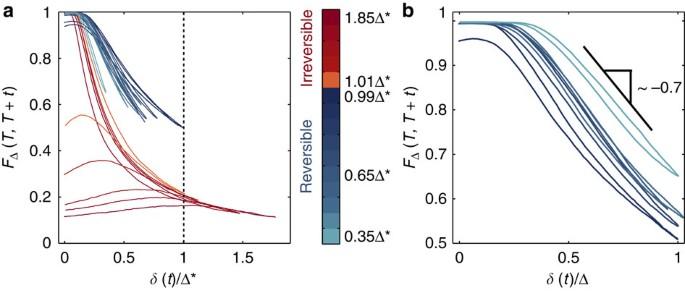Figure 2: Instantaneous fidelity loss over a cycle. (a) Instantaneous fidelity functionFΔ(T,T+t) plotted as a function of the rescaled instantaneous displacementδ(t)/Δ* for all the driving amplitudes. Again, the colour codes for the driving amplitude Δ. (b) Instantaneous fidelity functionFΔ(T,T+t) plotted as a function of the rescaled instantaneous displacementδ(t)/Δ in the reversible regime Δ<Δ*. For sake of clarity, only half of the experiments below the transition is displayed. The fidelity decays asymptotically as approximately −0.7δ(t)/Δ, which demonstrates that the emulsion self-organizes differently for each driving amplitude. Figure 2: Instantaneous fidelity loss over a cycle. ( a ) Instantaneous fidelity function F Δ ( T , T + t ) plotted as a function of the rescaled instantaneous displacement δ ( t )/Δ* for all the driving amplitudes. Again, the colour codes for the driving amplitude Δ. ( b ) Instantaneous fidelity function F Δ ( T , T + t ) plotted as a function of the rescaled instantaneous displacement δ ( t )/Δ in the reversible regime Δ<Δ*. For sake of clarity, only half of the experiments below the transition is displayed. The fidelity decays asymptotically as approximately −0.7 δ ( t )/Δ, which demonstrates that the emulsion self-organizes differently for each driving amplitude. Full size image For Δ<Δ* (blue curves), and δ ( t )/Δ*<<1, almost no particle escapes its initial Voronoï cell, and F Δ ( T , T + t ) hardly deviates from 1. For higher displacements, F Δ ( T , T + t ) decays linearly with δ ( t ) until t = T /2. Then starts the echo process, the direction of the flow is reversed and the system should retrace its steps back. As expected, F Δ ( T , T + t ) increases, linearly again, as δ ( t ) goes back to zero. However, in agreement with Fig. 1f , the dynamics is not fully reversible and the final value F Δ ( T ,2 T )=(Δ) is slightly smaller than 1, see Fig. 2b . Looking now at the variations of the instantaneous fidelity with δ ( t )/Δ in Fig. 2b , we readily note that the decay rate of the fidelity depends on the driving amplitude and decreases as Δ −1 . From this observation we infer a pivotal result: the conformation of the droplets, at the beginning of a cycle, is a function of the overall driving amplitude. In other words the emulsion self-organizes when periodically driven. We now consider the case of the higher amplitudes. For Δ>Δ* (red curves in Fig. 2a ), the variations of F Δ ( T , T + t ) are markedly different. During the first half of the cycle, F Δ ( T , T + t ) hardly depends on the driving amplitude: the fidelity decays rapidly and almost all the droplets rearrange. At the onset of flow reversal, some of the rearrangements are suppressed by the reversible dynamics and the fidelity increases. However, approaching the end of the cycle the droplets no longer manage to retrace their steps back anymore, and the fidelity decays again to reach a small (Δ) value. Importantly, in this limit, the system self-organizes into a state that does not depend on the driving amplitude anymore. Self-organization has been already demonstrated in a minimal model for periodically sheared suspensions introduced by Corté et al. [10] This model relies only on two-body contact interactions to account for the transition from a reversible to an irreversible state reported in refs 6 , 10 . In this model, the macroscopic reversibility on periodic shear was shown to correspond to the existence of many accessible absorbing states where the particles do not interact at all in the course of the cycles. Here we have described another possible scenario. Even for Δ<Δ* where the dynamics is reversible, the particles strongly interact. A macroscopic fraction of the droplets rearrange even for the smallest driving amplitudes ( Fig. 2a ). The instantaneous position of the individual droplets is not trapped inside an absorbing state. The phenomenology that we observe is actually similar to that found in soft solids close to the onset of plastic flows [5] , [8] . The existence of reversible ‘plastic’ events is a generic feature of dry grains, concentrated emulsions and suspensions interacting elastically when periodically driven below their yield stress [4] , [8] , [18] . We have shown above that: (i) the loss of fidelity results from a non-equilibrium phase transition and (ii) this collective phenomenon is associated to the self-organization of the droplets below the reversibility threshold. We now provide an explicit connection between these two findings and shed light on the nature of the self-organization process. Geometrically protected reversible states Looking at two instantaneous snapshots of the droplets below and above Δ* ( Fig. 3a,b , respectively), one clearly notices that the spatial structure of the emulsion strongly depends on the driving amplitude. The droplets fill the channel in a more homogeneous fashion when undergoing reversible trajectories. To go beyond this qualitative observation, we have plotted the variations of the (strobed) radial distribution function g ( r ) at the beginning of each cycle, for the different driving amplitudes shown in Fig. 3c . We also show the radial distribution corresponding to the initial conditions common to all the experiments, the highest curve as shown in Fig. 3c . In the initial state, g ( r ) is characterized by a strongly peaked value at r = a , which is characteristic of the steric repulsion between hard discs. Again, the droplets are non-deformed by the flow. A second narrow peak at r =2 a suggests that the droplets experience short-range attractive interactions. The position of the droplets loses any correlation above r =2 a . This structure is analogous to that found in confined fluidized beds made of rigid discs [19] , which demonstrates that the effective attractive interactions between the droplets do not result from any physicochemical adhesion force, but solely stem from hydrodynamic interactions. 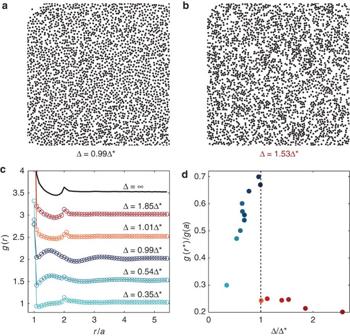Figure 3: Structural self-organization. (a) Snapshot of an emulsion shaken at Δ=0.99Δ* in the reversible regime,φ=0.37. (b) Snapshot of an emulsion shaken at Δ=1.53Δ* in the irreversible regime,φ=0.36. Note that the area fraction in (a,b) is quasi identical. (c) Strobed radial distribution functiong(r) for different driving amplitudes Δ. For sake of clarity, the curves are shifted vertically by a 0.5 constant value. A sharp change in the structure occurs at Δ*. Above Δ the structure of the emulsion does not depend on Δ any longer and remains identical to the one found in the initial state common to all the experiments (black curve). (d) Ratio of the fraction of droplets separated by a distancer*=1.5ato the fraction of droplets in close contact,g(r*)/g(a), plotted versus Δ/Δ*. A clear discontinuity occurs at Δ=Δ*, revealing a first-order structural transition. Figure 3: Structural self-organization. ( a ) Snapshot of an emulsion shaken at Δ=0.99Δ* in the reversible regime, φ =0.37. ( b ) Snapshot of an emulsion shaken at Δ=1.53Δ* in the irreversible regime, φ =0.36. Note that the area fraction in ( a , b ) is quasi identical. ( c ) Strobed radial distribution function g ( r ) for different driving amplitudes Δ. For sake of clarity, the curves are shifted vertically by a 0.5 constant value. A sharp change in the structure occurs at Δ*. Above Δ the structure of the emulsion does not depend on Δ any longer and remains identical to the one found in the initial state common to all the experiments (black curve). ( d ) Ratio of the fraction of droplets separated by a distance r *=1.5 a to the fraction of droplets in close contact, g ( r *)/ g ( a ), plotted versus Δ/Δ*. A clear discontinuity occurs at Δ=Δ*, revealing a first-order structural transition. Full size image In the small amplitude regime, Δ<<Δ*, the structure of the suspension is hardly modified. However, as Δ is further increased, the static structure of the emulsion self-organizes: the sharp peaks at r = a and r =2 a decrease while another structure emerges. The radial distribution displays an additional set of marked oscillations, revealing a structure analogous to a soft-sphere liquid at equilibrium, with a first wider peak located at r *~1.5 a regardless of the driving amplitude. As Δ approaches Δ*, the spatial correlation of this liquid-like structure increases up to distances as large as 7 particle diameters, see Supplementary Fig. 2 . Conversely, above Δ*, self-organization does not operate anymore and the emulsion weakly deviates from its initial conformation. The abrupt drop of the fidelity at Δ* coincides with a discontinuous structural change ( Fig. 3d ). This observation together with the superposition of two different marked structures below Δ* confirm a first-order phase-transition scenario, and suggests that the system undergoes a dynamical phase separation. We now provide a clear demonstration of this hypothesis. In Fig. 4a–c we show instantaneous conformations of the local fidelity field (see Supplementary Movies 4–6 for the corresponding strobed movies). Each Voronoï cell, defined at the beginning of the cycle, is coloured in blue when associated with a particle that retraces its step back to the very same cell at the end of the cycle. The cell is coloured in orange otherwise. At small amplitudes, Δ<<Δ*, clusters composed of very few irreversible events are dilute in a sea of reversible ones, see Fig. 4a . As Δ approaches Δ*, Fig. 4b , both the typical size and the number of those irreversible transient clusters increases, thereby inducing the fidelity decay as observed in Fig. 1f . The relation between the fidelity loss and the structural properties of the emulsion can now be clearly established. Using these fidelity maps, we plot in Fig. 4a,b the radial distribution function of the particles living in the reversible (resp. irreversible) region only. As the driving increases, the spatial structure in the irreversible regions remains unchanged. This structure corresponds to a hard-disc gas with attractive interactions as in the initial (homogeneous) state of the experiment. In contrast, in the reversible regions the droplets self-organize to form a soft-repulsive-disc structure. At the onset of the fidelity loss, the extent of translational order is maximal, thereby maximizing the typical distance between the neighbouring particles. The instantaneous conformation of the suspension is biphasic: two fluids having different structures coexist in two separated phases. This picture no longer holds above Δ* ( Fig. 4c ). All the particles then contribute in the same fashion to the average structure. The emulsion retains its initial spatial ordering, and the strong agitation impedes phase separation. Most of the particles undergo irreversible trajectories, and only a minute fraction of the Voronoï cells are associated with reciprocal motion. 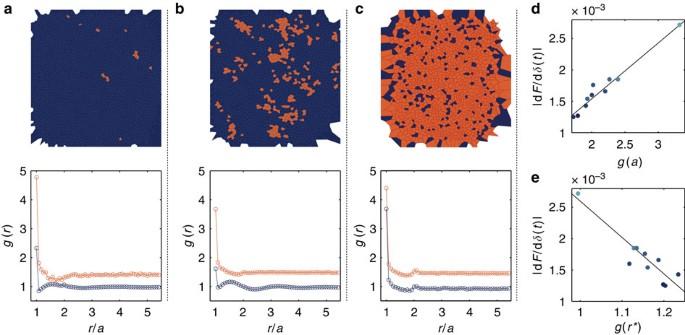Figure 4: Reversible-to-irreversible transition as a phase separation process. (a) Top: snapshot of the instantaneous fidelity field for Δ=0.54Δ*. Each Voronoï cell is coloured in blue when associated with a particle that retraces its steps back in the very same cell at the end of the cycle. The cell is coloured in orange otherwise. Bottom: strobed radial distribution functiong(r) computed in the reversible (resp. irreversible) cells. Same colour code. (b,c) Same plots as in (a) for Δ=0.99Δ* and Δ=1.53Δ*, respectively. The irreversible populations display a structure akin to a hard-attractive-disc fluid for all the driving amplitudes. Oppositely, the structure in the reversible regions depends on Δ. Below Δ*, the droplets self-organize to form clusters having a structure similar to a hard-attractive-discs liquid living in a sea of a soft-repulsive-discs liquid. For Δ≲Δ*, the correlation length of the translational order is maximal. The typical distance between neighbouring particles is maximal as well. Above Δ*, the instantaneous structure is homogeneous. Only a minute fraction of the droplets return stochastically into their initial Voronoï cell. (d) Slope of the linear part of the instantaneous fidelity decay |dFΔ(T,T+t)/dδ(t)|, plotted as a function of the fraction of particles in close contactg(a) (seeFig. 2b). The error bars corresponding to the standard deviation on the fit of |dFΔ(T,T+t)/dδ(t)| are smaller than the marker size. (e) Slope of the linear part of the instantaneous fidelity decay |dFΔ(T,T+t)/dδ(t)|, plotted as a function of the fraction of particles at a distancer*,g(r*). The error bars corresponding to the standard deviation on the fit of |dFΔ(T,T+t)/dδ(t)| are smaller than the marker size. Same colour code as in all the previous plots. Figure 4: Reversible-to-irreversible transition as a phase separation process. ( a ) Top: snapshot of the instantaneous fidelity field for Δ=0.54Δ*. Each Voronoï cell is coloured in blue when associated with a particle that retraces its steps back in the very same cell at the end of the cycle. The cell is coloured in orange otherwise. Bottom: strobed radial distribution function g ( r ) computed in the reversible (resp. irreversible) cells. Same colour code. ( b , c ) Same plots as in ( a ) for Δ=0.99Δ* and Δ=1.53Δ*, respectively. The irreversible populations display a structure akin to a hard-attractive-disc fluid for all the driving amplitudes. Oppositely, the structure in the reversible regions depends on Δ. Below Δ*, the droplets self-organize to form clusters having a structure similar to a hard-attractive-discs liquid living in a sea of a soft-repulsive-discs liquid. For Δ ≲ Δ*, the correlation length of the translational order is maximal. The typical distance between neighbouring particles is maximal as well. Above Δ*, the instantaneous structure is homogeneous. Only a minute fraction of the droplets return stochastically into their initial Voronoï cell. ( d ) Slope of the linear part of the instantaneous fidelity decay |d F Δ ( T , T + t )/d δ ( t )|, plotted as a function of the fraction of particles in close contact g ( a ) (see Fig. 2b ). The error bars corresponding to the standard deviation on the fit of |d F Δ ( T , T + t )/d δ ( t )| are smaller than the marker size. ( e ) Slope of the linear part of the instantaneous fidelity decay |d F Δ ( T , T + t )/d δ ( t )|, plotted as a function of the fraction of particles at a distance r *, g ( r *). The error bars corresponding to the standard deviation on the fit of |d F Δ ( T , T + t )/d δ ( t )| are smaller than the marker size. Same colour code as in all the previous plots. Full size image To further emphasize the relation between the dynamical and the structural properties of the emulsion, we now show that the number of particles that escape their initial Voronoï cell in the course of a cycle is set by the typical distance between the neighbouring droplets. To do so, we plot the decay of the instantaneous fidelity per displacement unit: |d F Δ ( T , T + t )/d δ ( t )| (slope of the straight lines in Fig. 2a ) as a function of g ( a ) and g ( r *), see Fig. 4d,e . When self-organization occurs, Δ<Δ*, the fidelity-decay rate increases linearly with g ( a ), which is the fraction of droplets in close contact. In contrast, this decay rate decreases with g ( r *), viz. as the fraction of droplets separated by a finite distance r *~1.5 a increases. In other words, pushing the droplets apart the escape rate from the initial Voronoï cells is restrained: macroscopic reversibility is geometrically protected by a structural self-organization. Irreversibility and memory loss We have hitherto investigated the dynamics of the emulsion in real space from a condensed matter perspective. To gain more physical insight on the origin of reversibility loss on periodic driving, we now sketch the trajectory of the system in its 2 N -dimensional phase space, black line in Fig. 5a . If the particles were to interact uniquely via (time-reversible) hydrodynamic interactions, this trajectory would be reciprocal. However, in an experiment, or in a numerical simulation, any minute non-time-reversible perturbation along the trajectory is expected to be amplified due to the chaotic nature of this many-body system [3] , [6] , [20] . As a result, the phase-space trajectory should separate into two different back and forth paths. Exploiting the invariance on time reparametrization of the hydrodynamic interaction, we can reverse the arrow of time along the first part of the cycle (red curve in Fig. 5a ). By doing so, the two half-trajectories are analogous to two different realizations of the system dynamics for initial conditions taken at t = T /2. The asymptotic separation between these two perturbed trajectories after a time t is measured by computing the metric distance in phase space between the conformations of the particles at times T /2− t and T /2+ t . We denote this distance by D ( t ). In Fig. 5b , D ( t ) is plotted as a function of the instantaneous mean displacement δ ( t ) for all driving amplitudes Δ. For Δ<Δ*, D ( t ) displays a clear exponential increase, which allows for measuring the largest Lyapunov exponent of the underlying chaotic dynamics. Above Δ*, the Lyapunov picture breakdown and the separation between the trajectories increases algebraically, see Fig. 5b inset. 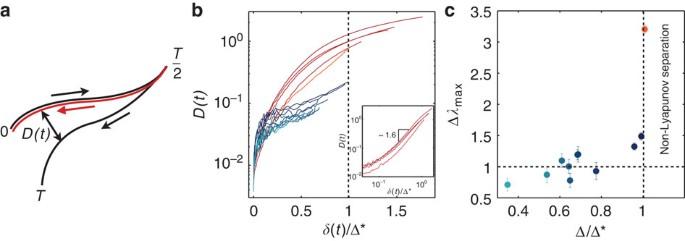Figure 5: Trajectories separation in phase space. (a) Sketch of the trajectory of the system in its 2N-dimensional phase space on periodic driving (black lines). These two paths differ due to the chaotic amplification of any minute non-time-reversible perturbation. Reversing the arrow of time along the first half of the cycle (red curve), these two trajectories are two different realizations of the system dynamics, for initial condition taken att=T/2. (b) Semi-log plot ofD(t) as a function ofδ(t)/Δ* for all the driving amplitudes. Same colour code as in the previous figures. Inset: log-log plot. Above Δ*, the separation is no longer exponential but algebraic. (c) Plot of Δλmaxas a function of Δ/Δ*, revealing memory loss at the onset of irreversibility. The error bars correspond to the standard deviation on the fit ofD(t). Figure 5: Trajectories separation in phase space. ( a ) Sketch of the trajectory of the system in its 2 N -dimensional phase space on periodic driving (black lines). These two paths differ due to the chaotic amplification of any minute non-time-reversible perturbation. Reversing the arrow of time along the first half of the cycle (red curve), these two trajectories are two different realizations of the system dynamics, for initial condition taken at t = T /2. ( b ) Semi-log plot of D ( t ) as a function of δ ( t )/Δ* for all the driving amplitudes. Same colour code as in the previous figures. Inset: log-log plot. Above Δ*, the separation is no longer exponential but algebraic. ( c ) Plot of Δ λ max as a function of Δ/Δ*, revealing memory loss at the onset of irreversibility. The error bars correspond to the standard deviation on the fit of D ( t ). Full size image Following ref. 21 , we expect reversibility to be lost when the chaotic amplification of the microscopic fluctuations causes the system to forget about its initial state in a time smaller than T /2, that is, over a mean displacement smaller than Δ. In more quantitative terms, we expect the fidelity to decay for λ max Δ~1, where the largest Lyapunov exponent λ max is defined as D ( t )~exp[ λ max δ ( t )] asymptotically. This hypothesis is confirmed by plotting the product λ max Δ as a function of Δ/Δ* in Fig. 5c . Below the onset of fidelity decay, the structural self-organization induces variations of λ max that almost exactly balance the increase in the drive amplitude: λ max Δ~1. Conversely, as Δ exceeds Δ*, the path memory is lost, λ max Δ>1 and the fidelity decays accordingly ( Fig. 5c ). As a last physical comment, we note that the scaling λ max ~1/Δ is the signature of the convergence towards an absorbing dynamics. Repeating echo protocols, the system evolves towards a phase-space region where λ max Δ~1 and where the trajectories are fully reversible ( F ~1). Hence, the strobed dynamics is frozen and the system cannot escape this absorbing region. Note, however, that these absorbing states refer uniquely to the strobed dynamics, as opposed to the scenario put forward in refs 10 , 13 where the dynamics is frozen along the entire trajectories. Again this situation is very different from that reported here. We can therefore conjecture that the transition towards irreversibility occurs when all the regions of phase space where λ max is small enough are either out of reach starting from a strongly shaken state or do not exist. The latter scenario is consistent with the long-range nature of the hydrodynamic interactions (~1/ r 2 decay in 2D [14] ), which strongly couples the entire population of particles regardless of their conformation. Taking advantage of a quantitative microfluidic experiment, we have demonstrated that periodic shaking results in the emergence of structural order in an ensemble of particles interacting in a time-reversible fashion. Unlike equilibrium systems, this geometric self-organization protects the macroscopic reversibility of the system and realizes a (non-equilibrium) Loschmidt-echo experiment. Even though our primary motivation was to gain a deeper insight into the collective dynamics of periodically driven systems, we anticipate this study to be of practical relevance. Hydrodynamic interactions in fine-tuned flows have recently been shown to be a potential means to programme-directed colloidal assembly [22] . Here we have demonstrated that even in the simplest possible flow field (a plug flow), hydrodynamic interactions can be put to work to induce spatial ordering in an emulsion. Over the last 5 years, much effort has been devoted to synthesizing non-spherical colloids in the 1–100 microns range, see, for example, refs 23 , 24 . Given our observations, using simple AC hydrodynamic actuation could be a powerful tool to trigger and tailor their self-assembly over massive scales, which until now has remained a major practical issue. Microfluidics The microfluidic device is a double-etched fused silica/quartz chip (Micronit Microfluidics), as sketched in Supplementary Fig. 1 . It consists of: (i) a conventional flow-focusing junction used to form monodisperse droplets, (ii) a dilution module made of an additional cross junction and (iii) two 0.5 cm × 5 cm channels. One of the two wide channels is used to transfer the polydisperse droplets produced in the transient regime of the drop emitter. The other one is used to perform the experimental observations, see, for example, Fig. 1a and Supplementary Movie 1 . The height of the flow-focusing and of the dilution modules is 11 μm while the two large channels are 27 μm high. The fluids are injected using three syringe pumps (Cetoni, Nemesys) connected to the three inlets of the device (inlets (1), (2) and (3) in Supplementary Fig. 1 ). Hexadecane is injected through (1) and the continuous phase (0.1 wt% SDS (Sigma), 0.2 wt% fluorescein (Sigma) in deionized water ) is injected both through inlets (2) and (3). The channel surfaces were cleaned in a UV/Ozone cleaner through the quartz surface prior to the experiments. As a result, both the glass and the quartz surfaces are highly hydrophilic, thereby preventing partial wetting of the walls by the dispersed phase). The area fraction Φ=0.36 is obtained by setting the flow rates as Q (1) =0.040 μl s −1 , Q (2) =0.140 μl s −1 and Q (3) =3 μl min −1 . The emulsion is periodically driven by imposing an oscillatory flow rate at the outlet (4). To impose the various values of Δ, the magnitude and period of the sinusoidal oscillations are set to values comprised between 0.02< Q <0.039 μl s −1 and 10< T <30 s, respectively. As expected, the variations of Δ are linear in Q and T . Prior to any experiment, the system is prepared by imposing a high amplitude sinusoidal oscillation ( Q =0.1 μl s −1 ) during several cycles. This protocol is chosen to set reproducible initial conditions. To make sure that the system is in a steady state, the image acquisition is performed after 1,000 cycles at the desired flow rate and period, and we systematically check that all the measured quantities are statistically stationary. The droplet positions are recorded over 150 (Δ>Δ*) or 700 cycles (Δ<Δ*). Imaging and particle tracking The device is mounted on a Nikon AZ100 upright microscope. A Basler Aviator av2300-25gm (4 megapixel, 8 bit) camera is used to record the movement of the droplets in a field of view of 2.70 mm × 2.03 mm at the centre of the main channel. The frame rate is set at 24 Hz. Image acquisition is performed using a custom direct-to-disk Labview code. The particles are detected to a one-pixel accuracy. The particle velocities are then computed using the Matlab version of the tracking software developed by Grier, Crocker and Weeks [25] . How to cite this article: Jeanneret, R. & Bartolo, D. Geometrically-protected reversibility in hydrodynamic Loschmidt-echo experiments. Nat. Commun. 5:3474 doi: 10.1038/ncomms4474 (2014).